Genomic analysis reveals selection for Asian genes in European pigs following human-mediated introgression The independent domestication of local wild boar populations in Asia and Europe about 10,000 years ago led to distinct European and Asian pig breeds, each with very different phenotypic characteristics. During the Industrial Revolution, Chinese breeds were imported to Europe to improve commercial traits in European breeds. Here we demonstrate the presence of introgressed Asian haplotypes in European domestic pigs and selection signatures on some loci in these regions, using whole genome sequence data. The introgression signatures are widespread and the Asian haplotypes are rarely fixed. The Asian introgressed haplotypes are associated with regions harbouring genes involved in meat quality, development and fertility. We identify Asian-derived non-synonymous mutations in the AHR gene that associate with increased litter size in multiple European commercial lines. These findings demonstrate that increased fertility was an important breeding goal for early nineteenth century pig farmers, and that Asian variants of genes related to this trait were preferentially selected during the development of modern European pig breeds. Thousands of years of selection on numerous traits in domesticated species such as dogs [1] , [2] , cows [3] and chickens [4] has led to a wide range of distinct phenotypes that are not (or only rarely) observed in the wild. Improvement of breeding practices, which involves making crosses between different breeds and even (sub)species, has greatly improved productivity in intensive farming systems. Examples include the white seed colour in rice, shown to originate from a single mutation that swept through different subspecies following hybridization [5] , and the yellow skin allele that is fixed in the majority of modern western chicken breeds originating from admixture with the Grey junglefowl [6] . Human-mediated introgression of alleles is likely to have played a major role in the genomic architecture of many modern domestic species, including pigs. The wild boar ( Sus scrofa ) originated ~4 million years ago in Southeast Asia and has since expanded its range over Eurasia, leading to the emergence of numerous geographically and genetically divergent populations [7] , [8] . The independent domestication of two of these populations in East Asia and western Eurasia led to distinct domesticated populations [9] , [10] , [11] . Hybridization and introgression between domestic pigs that originated from highly divergent wild populations has resulted in modern genomes that possess a mosaic of different haplotypes [12] , [13] . Although some gene flow may have taken place before the nineteenth century, it was certainly extremely rare given the geographic distance between Asia and Europe, and the lack of any historical records describing the importation of Asian breeds into Europe before the nineteenth century (or vice-versa). Mitochondrial studies have suggested that the introgression was mostly female driven [12] and the introduction of Asian pigs into Europe at the onset of the Industrial Revolution in the late eighteenth and early nineteenth centuries has been particularly well documented [14] , [15] . In parallel with increasing intensification of farming at that time, British pig breeders sought to improve productivity of the local breeds, and did so, in part, by importing Chinese pigs. Chinese pigs were renowned for having great mothering characteristics, superior meat quality, strong resistance to diseases, better adaptation to living in sties and producing larger litters (>15 live born young). The selection for specific traits in European pig breeds has resulted in multiple selective sweeps in the genome of domesticates [16] . As European pig breeders deliberately introgressed Asian haplotypes into European local breeds, it is expected that the origin of haplotypes for which evidence of selection exists often stems from Asian introgression. Known examples include the EDNRB , IGF2 and KITLG regions [17] , [18] , [19] , all of which the identified variants have considerable effect on the phenotypes. Interestingly, the selection criteria shifted through time. When Asian lines were first introgressed into European pigs, fatness was selected for, although now leanness is preferentially selected. The Large White (LW) breed is one of most widely used breeds in commercial pig production and originated in the United Kingdom in the late nineteenth century. The breed is renowned for high growth rate, desirable carcass lean meat percentage and a desirable feed to body weight conversion ratio, but also for large litters, heavy milk production and great mothering characteristics. As LW is thought to have a hybrid origin, some of these traits are potentially the result of selected Chinese haplotypes. Because of deliberate introduction of Asian germplasm into European pigs and subsequent intensive artificial selection, Asian haplotypes in LW genomes are expected to be non-randomly distributed, but rather to be overrepresented in regions that contain genes or regulatory elements that are linked to traits relevant for production. Here we test this hypothesis and identify specific gene variants bred into European pigs involved in key production traits. More specifically, we interrogated the genomes of LW pigs to reveal patterns of introgressed and selected haplotypes, to unravel the genomic consequences of human-mediated hybridization and artificial selection. Evidence of introgression We identified haplotypes in the LW pigs that were identical by decent (IBD) with individuals from both the original source of domestication, the European wild boars (EUWB), and the source of introgression, the Asian domestic group (ASDom, Fig. 1 ). 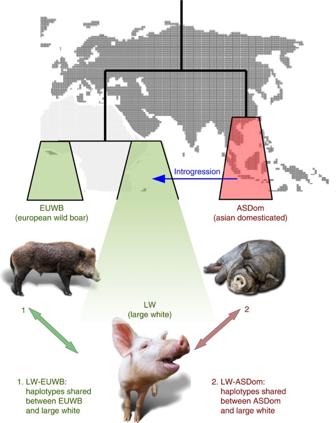Figure 1: Experimental setup for the introgression detection. Arrows indicate the comparisons between groups that are used for the IBD detection. Individuals from the LW breed are used for all pairwise comparisons with individuals from two geographical and functional groups: EUWB and ASDom. The blue arrow indicates the human-mediated introgression from ASDom in to LW. Individuals from different locations in Europe were used to represent the source of domestication, whereas individuals from three different Asian breeds were used to represent the pool of putative introgressed haplotypes (see Supplementary Table 1 and Supplementary Methods for details). Average genetic differentiation (Fst, as defined by Weir and Cockerham [20] ) between the LW and ASDom was 0.33 (s.d. 0.23, s.e. 0.0008), while the average Fst value between LW and EUWB was 0.16 (s.d. 0.17, s.e. 0.0006). These results show that the genomes of the LW pigs still share greater similarity with their EUWB ancestors than with ASDom. We used an other independent method to further verify the existence of gene flow between ASDom and LW after lineage divergence between Asian and European Sus scrofa (D-statistics [21] , see Methods). We computed this statistic for each possible trio between (LW, ASDom and EUWB), and (LW, EUWB, ASDom) so that a significantly negative D ( Z <−4) imply admixture between ASDom and LW. Our results demonstrate that all LW individuals possess roughly an equal degree of admixture with Asian pigs over their entire genomes, reflecting the human-mediated hybridization with Asian domestics in the late eighteenth and early nineteenth century ( D =−0.083±0.015, Z =−20). Figure 1: Experimental setup for the introgression detection. Arrows indicate the comparisons between groups that are used for the IBD detection. Individuals from the LW breed are used for all pairwise comparisons with individuals from two geographical and functional groups: EUWB and ASDom. The blue arrow indicates the human-mediated introgression from ASDom in to LW. Full size image Introgression mapping To infer whether a region was introgressed in multiple individuals, we calculated the frequency of all LW haplotypes that were of Asian or European origin for each bin of 10,000 bases in the genome. The relative fraction of Asian versus European haplotypes in the LW group is expressed as relative IBD (rIBD). Asian haplotype frequency in the LW population, for a given locus, ranged from 0.7 (where 1 indicates all haplotypes are ASDom and none are EUWB) to −1 (all haplotypes are IBD with EUWB, Fig. 2a ). The majority of the genome displays more similarity with the EUWB than with the Asian domesticated pigs. Despite this, every chromosome contained regions in which the signal for Asian ancestry was stronger than the European signature. A cutoff of two s.d. from the mean in the Z-transformed rIBD distribution allowed us to identify regions, which spans ~1.3% of the genome of LW pigs, that were likely to be of Asian origin ( Fig. 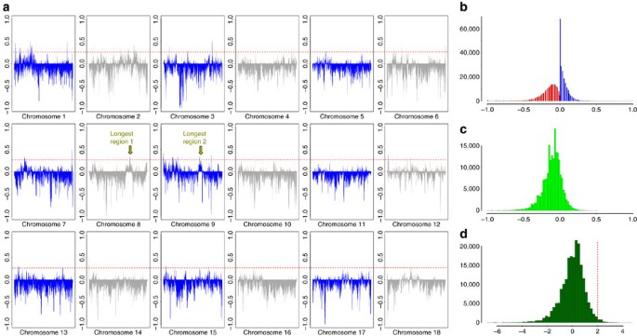Figure 2: Distribution of regions in the genome where the LW contain introgressed haplotypes from ASDom. (a) Thexaxis shows the full length of all chromosomes, and theyaxis represents the relative frequency of LW haplotypes IBD with ASDom or EUWB, ranging from 1 (all haplotypes are IBD with ASDom, and none with EUWB) to −1. The two longest regions of consecutive introgression are indicated with arrows. (b) Distribution of the relative proportion of IBD haplotypes in LW and the EUWB (green, IBDEUWB, 0 to −1) or ASDom (blue, IBDASDom, 0 to 1) in bins of 10 Kbp. (c) Distribution of the rIBD scores for the LW haplotypes (rIBD=IBDEUWB–IBDASDom). (d)Z-transformed distribution of rIBD. 2c,d and Supplementary Table 2 ). Figure 2: Distribution of regions in the genome where the LW contain introgressed haplotypes from ASDom. ( a ) The x axis shows the full length of all chromosomes, and the y axis represents the relative frequency of LW haplotypes IBD with ASDom or EUWB, ranging from 1 (all haplotypes are IBD with ASDom, and none with EUWB) to −1. The two longest regions of consecutive introgression are indicated with arrows. ( b ) Distribution of the relative proportion of IBD haplotypes in LW and the EUWB (green, IBDEUWB, 0 to −1) or ASDom (blue, IBDASDom, 0 to 1) in bins of 10 Kbp. ( c ) Distribution of the rIBD scores for the LW haplotypes (rIBD=IBDEUWB–IBDASDom). ( d ) Z -transformed distribution of rIBD. Full size image This introgression pattern is probably the result of a combination of drift and selection. In contrast to dogs, where selection seems to have acted on a relatively small number of loci with large effects [1] , [2] , the introgression signal in the pigs is found at many loci, and the putatively selected Asian haplotype is rarely fixed. This pattern suggests that selection on Asian haplotypes, if present, mostly involved complex multi-genic traits or genes influencing traits selected in opposing directions. A high rIBD signal in our analysis refers to a region that contains predominantly introgressed haplotypes, but this does not imply that the introgressed haplotypes are identical or similar. Regions that contain more Asian haplotypes just by chance, but have not been under selection, could result in a high rIBD signal. We used an extended haplotype homozygosity test [22] to check for extended haplotypes in the LW population and compared the integrated haplotype score (iHS) signal with our rIBD values. This way, we can distinguish between regions that contain multiple Asian haplotypes and regions that contain one or few particular elongated Asian haplotypes. We inferred a significant correlation between rIBD and integrated haplotype score (iHS) in bins of 500 kb over the full genome ( Supplementary Fig. 1a ). To check whether the extended haplotype homozygosity in the LW pool was specific for the breed or observed in more European breeds, we contrasted the LW signal with a reference pool of other European commercial pigs ( Supplementary Fig. 1b,c ). Genome-wide patterns of introgression On a genome scale, many of the genes located within the regions where the LW pigs share more haplotypes with ASDom than with EUWB (σZrIBD≥2), are associated with commercial traits such as meat quality ( DNMT3A , SAL1 , ME1 , IGF2BP1 ), fertility ( PGRMC2 , KIF18A CDK20 , AHR ) and development ( NRG1 , AHR , Supplementary Table 2 ), although no significant enriched Gene Ontology (GO) term was found. Gene-dense regions on chromosome 1 and 2 display a high rate of alternating ASDom and EUWB haplotypes. For instance, the regions containing the CDK20 and SAL1 genes, which both have been associated with reproduction traits [23] , [24] , are only 10–20 kb long. These short tracts of shared haplotypes either indicate a high recombination frequency (corroborated by the recombination map for pig [25] ), a more temporally distant hybridization episode and/or favourable European haplotypes surrounding these genes that could lead to positive selection on recombinant haplotypes. The recombination landscape in Sus scrofa is known to be highly heterogeneous, and this probably results in an unequal distribution of haplotype length [26] . Longer Asian haplotypes will be found in regions of low recombination and therefore the introgression signal is easier to identify in regions with a low recombination rate. Longest regions of introgression Chromosomes 8 and 9 contain the largest consecutive regions of inferred introgression in the LW genomes (defined as regions where rIBD>0). To check whether the extended haplotype homozygosity in the LW pool was specific for the breed or observed in more European breeds, we contrasted the LW signal with a reference pool of other European commercial pigs with the Rsb statistic [27] ( Supplementary Fig. 1b,c ). This analysis demonstrates that the region of introgression on chromosome 8 contains a stronger extended haplotype homozygosity (EHH) signal in the reference panel, and that the region on chromosome 9 contains a particularly strong signal in the LW population. We used two independent methods, D -statistics and Fst, to support the detected introgression in these regions in the LW ( Fig. 3a–e ). To show that divergence between LW and ASDom was reduced in the introgressed regions, we calculated Fst for these regions separately. The Fst between ASDom and the LW was lower in both introgressed regions than between EUWB and LW ( Fig. 3c-e ), thereby supporting the signal of Asian introgression (high rIBD). The D -statisctics for the regions on chromosome 9 was lower than the genome-wide average, which corroborated our rIBD analysis ( Fig. 3b ). The region on chromosome 8 shows a wide distribution, indicating that some LW haplotypes contain the Asian signature, while others do not. Inconsistent clustering of European haplotypes within an Asian clade at this locus supports this hypothesis ( Supplementary Fig. 2 ). Curiously, the ~4 Mb sequence shows a clear signal of introgression, although a large part of the region is devoid of annotated genes. As this part of the genome has a relatively low recombination frequency [25] , the region may extend considerably beyond the position of the actual favourable allele that has been selected for, due to genetic hitch-hiking and the short time since introgression. Alternatively, drift could have resulted in the presence of Asian haplotypes in this region. The PGRMC2 gene, coding for the progesterone receptor, lies within the highest peak of Asian haplotypes in that region. Progesterone is an important hormone involved in female reproduction and maternal behaviour [28] , traits that Asian pigs have been selected for extensively. Therefore, the Asian haplotype containing the PGRMC2 gene could be associated with higher reproductive success in LW pigs and may have been subjected to selection pressure as a result. The Rsb signal suggest that in other European breeds, the proportion of Asian haplotypes is even higher for this locus ( Supplementary Fig. 1b,c ). We used genotype data from the Illumina Porcine 60K iSelect beadchip [29] for an additional 5,143 pigs from three European commercial lines to screen allele frequencies in this region. Two genetic lines have been selected for reproductive traits since the establishment of the lines (A and B), and one line for finishing traits (C). The SNP alleles in this 4-Mb region show a clear difference between the two reproduction-associated lines and the growth-associated line ( Supplementary Fig. 3 ). These findings could indicate that the Asian haplotypes in this region are associated with fertility, but further analyses are needed to support this hypothesis. 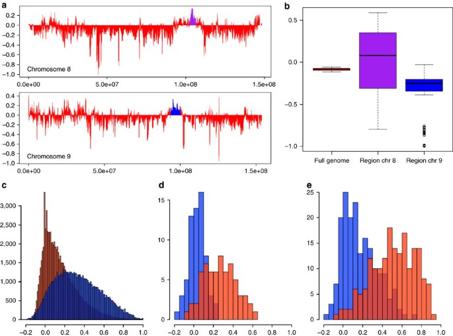Figure 3: Levels of differentiation between LW and ASDom or EUWB in regions of introgression. (a) Relative introgression fraction (rIBD) over the full length of chromosome 8 and 9. The longest regions of introgression are indicated with purple and blue. (b) Boxplot ofD-statistics for the full genome (red) and the two longest regions of introgression as indicated inaon chr8 (purple) and chr9 (blue). The minimum, first quartile, median, third quartile and maximum are indicated with the box and whiskers with outliers >1.5*IQR.D-statistics are computed for each possible trio with LW=P1, ASDom=P2 and EUWB=P3, with the SumatranS. scrofaas outgroup (O) resulting in 378 trios. (c–e) Distribution of Fst between LW-ASDom (blue) and LW-EUWB (red) in bins of 10 Kbp. The left histogram shows the Fst distributions based on the full genome (c), and the other two show the Fst distribution for the regions of introgression on chr8 (d) and chr9 (e). Figure 3: Levels of differentiation between LW and ASDom or EUWB in regions of introgression. ( a ) Relative introgression fraction (rIBD) over the full length of chromosome 8 and 9. The longest regions of introgression are indicated with purple and blue. ( b ) Boxplot of D -statistics for the full genome (red) and the two longest regions of introgression as indicated in a on chr8 (purple) and chr9 (blue). The minimum, first quartile, median, third quartile and maximum are indicated with the box and whiskers with outliers >1.5*IQR. D -statistics are computed for each possible trio with LW=P1, ASDom=P2 and EUWB=P3, with the Sumatran S. scrofa as outgroup (O) resulting in 378 trios. ( c – e ) Distribution of Fst between LW-ASDom (blue) and LW-EUWB (red) in bins of 10 Kbp. The left histogram shows the Fst distributions based on the full genome ( c ), and the other two show the Fst distribution for the regions of introgression on chr8 ( d ) and chr9 ( e ). Full size image Introgression at the AHR locus The 6.8-Mb region on chromosome 9 has a large proportion of LW haplotypes that are nearly identical to two haplotypes found in the Asian Jianquhai breed ( Supplementary Fig. 2 ). Among the genes in this region of putative Asian introgression are multiple members of the TWIST gene family, transcription factors known to be involved in a variety of processes, including embryonic development [30] . The highest introgression peak in this region contains the AHR gene that has previously been associated with female reproductivity [31] . Originally, the AHR gene has been identified as mediator of xenobiotic-induced toxicity [32] , [33] . AHR has been shown not only to be involved in the response to toxicity but also to be associated with fertility in mammals [34] , [35] . The AHR gene seems to play an important role in the female reproductive system at multiple levels [31] . In pigs, expression of AHR during the oestrous cycle and putative involvement of AHR in the regulation of reproduction has been observed [36] , [37] . Furthermore, polymorphisms in human are known to occur predominantly in exon 10, which contains an important transactivation domain [38] . We screened this gene in pigs for non-synonymous mutations and identified four non-synonymous mutations in exon 11 of the AHR gene, which corresponds to exon 10 of the human AHR gene. The variants of Asian origin were all in strong linkage disequilibrium. As the AHR is a strong candidate gene for which Asian variants have been selected since introgression during the Industrial Revolution, we examined this gene further (see Methods). The iHS signal within the LW population is strongest for the AHR locus. The fact that the Rsb signal is also strong in the LW compared with other European breeds, indicates that the Asian haplotypes at the AHR locus were never fixed in the ancestral population that led to current commercial breeds, because the frequency and iHS signal differs between breeds ( Supplementary Fig. 1b,c ). We used an additional method to screen for selection, nSL, that has recently become available and should be robust to variation in recombination rate [39] . We averaged the rIBD, the nSL statistic and the corrected iHS P -value over bins of 500 kb for chromosome 9 (see Supplementary Fig. 4a–c ). All three statistics contain a high signal at the previously identified region on chromosome 9 that also contains the AHR gene. We show that the haplotype containing the ancestral allele at the AHR locus is more persistent than haplotypes containing the derived allele at this locus ( Supplementary Fig. 4d–f ). A survey of wild boar populations and four other Sus species for these loci revealed that the ancestral haplotype is homozygous in all closely related Sus species, and at high frequency in Asian domesticated pigs and European breeds. However, only derived haplotypes were found in European wild boar and the ancestral type was present only at a low frequency in Asian wild boars. This suggests a history of selection for the ancestral state in domestics, after the derived state reached high frequency in the wild populations. Effect of Asian haplotypes at the AHR locus To examine the effect of the amino acid changes in the AHR protein on reproductive success, we used genotype data from the Illumina Porcine 60K iSelect beadchip [29] for the same 5,143 pigs from three European commercial purebred lines for which estimated breeding values (EBV) for the total number of piglets born (TNB) were available. We extracted genotypes for those markers that fell within the region of high introgression (rIBD>2). The AHR gene was the only annotated gene in this selected part of the genome. Either Asian or European heritage was assigned to the 60K haplotypes for these 5,143 commercial pigs at the AHR locus, based on our re-sequenced individuals and confirmation in the lab (see Methods). Haplotypes containing the Asian AHR variants had a significant effect on the EBV for total number born over all three lines (EBV–TNB 0.162, s.e. 0.04, P <0.0001, Table 1 ). Although the EBV–TNB can be rather different between different lines, within-line effects of the Asian allele were also estimated. A difference of 0.1 in EBV equates to a difference of 0.1 piglets born. As total number of piglets born is a complex multi-locus trait, an increase of 0.16 piglets born (across all three breeds) is substantial in the current breeding industry. If the costs of maintaining a sow on a farm are spread over a larger number of piglets being weaned from that sow, the marginal cost reduction of producing a finishing pig is just over 3 euros per extra piglet [40] , that is, 2% of that total. Even though we cannot rule out that the effect could be due to some extended haplotypes covering other genes in the region, these details in combination with known literature contribute to AHR as the strongest candidate gene. Table 1 Estimated breeding values for total number born per line for haplotypes containing Asian or European alleles at the AHR locus. Full size table Interestingly, the AHR locus is an example of selection on the ancestral state that was either lost or never present in the European wild population. Re-introduction of the variants by introgression of Asian haplotypes and the positive effect of these alleles on litter size contributed to the high frequency of Asian haplotypes at the AHR locus in the current population. As the AHR gene seems to be involved in multiple life history traits, it could very well be that some long-term balancing selection acted on the alleles. The AHR gene is involved in multiple traits and during ever-changing adaptation to, for example, different environments, some alleles might be more desirable than others under different circumstances [41] . The significant association between the Chinese haplotypes and an increased EBV for total number born, which in our opinion is a strong independent indication for selection, in combination with the selection sweep results provide convincing evidence for the AHR locus to have been under selection after introgression. Similar examples of selection on Asian haplotypes in European pigs exist in literature, such as the signals of selection associated with coat colour [42] , ear morphology [17] and increased lean content [19] . The evidence presented here demonstrates how crossing of divergent populations may shape the variation on a genome-wide scale in populations. The introduction of Asian haplotypes into European breeds in the late eighteenth and early nineteenth centuries [8] , [9] and consecutive selection for desired traits in these breeds thereby provides a robust, historically documented model system for these instances. We identified numerous genomic regions where Asian haplotypes were introgressed into a larger European background, including the AHR locus. The AHR gene has been known to be involved in reproduction [34] , [35] , [36] , [37] , and our study corroborates that earlier report by demonstrating a significant increase in litter size in European commercial pigs that possess the Asian haplotype. Our findings provide a unique insight into the genomic haplotype patterns resulting from breeding practices from first domestication until the intensive breeding industry we know today. The observed introgression pattern is a combination of drift and selection, and detailed analyses such as those demonstrated for the AHR locus will shed more light onto the importance of other introgressed Asian haplotypes on signatures of selection in modern pig breeds. Sample collection and DNA preparation Blood samples were collected from a total of 70 individual, wild and domesticated S. scrofa . Among these individuals were 2 wild boars from Sumatra, 8 Asian wild boars from China and Japan, 18 EUWB from the Netherlands, France, Switzerland, Greece and Italy, 13 Asian domesticated pigs from the Meishan, Jianquhai and Xiang breeds and 29 European domesticated pigs from the Duroc, Hampshire, Pietrain, Landrace and LW breeds. DNA was extracted from the blood samples with the use of the QIAamp DNA blood spin kit (Qiagen Sciences) and checked for quality and quantity on the Qubit 2.0 fluorometer (Invitrogen). Library construction for the re-sequencing was performed with 1–3 μg of genomic DNA according to the Illumina library prepping protocols (Illumina Inc.) and the insert size varied from 300 to 500 bp. Sequencing was performed on 1–3 μg of genomic DNA with the 100 paired-end sequencing kit for all samples. Single nucleotide polymorphism (SNP) genotyping was performed on the Illumina Porcine 60K iSelect Beadchip [26] . DNA from all individuals was diluted to 100 ng μl and genotyped according the IlluminaHD iSelect protocol. Data was analysed using Genome Studio software (Illumina Inc.). Alignment and variant calling All individuals were re-sequenced with the Illumina paired-end sequencing technology (Illumina Inc.) to ~10 × depth of coverage (details in Supplementary Table 1 ). The read pairs were trimmed to have a minimum phred quality >20 over three consecutive bases, while each mate should have a minimal size of 45 bp after trimming. Alignment was performed with Mosaik Aligner (V. 1.1.0017) with the unique alignment option to the Porcine reference genome build 10.2. Variants were called using Samtools mpileup 0.1.12a (r862). The alternative allele should be covered at least two times to call an SNP and INDELS were excluded. VCFtools was used for filtering for a genotype quality of >20, a minimum read depth of 7 × and a maximum read depth of twice the average read depth. For the list of all those sites that were heterozygous or non-reference within at least one individual, genotyping was performed with Samtools mpileup for all 70 individuals to create a matrix containing an unbiased representation of the variation present in the samples. Homozygous reference alleles were also included in the matrix at this stage, and only those sites that were covered ≥4 × in all individuals were included, resulting in 2,377,607 markers. Pairwise IBD detection The matrix of 70 individuals genotyped for 2,377,607 positions in the genome served as input for the IBD detection pipeline. All individuals were phased with the fastPhase function in Beagle version 3.3.2. Pairwise shared haplotypes were extracted with the Beagle fastIBD function as described by Browning and Browning [43] . Phasing and IBD detection was executed ten times independently and identified IBD tracts were merged from all ten runs, as suggested by the authors. Partially overlapping runs were extracted and the IBD runs with the highest probability scores were added to the pool of IBD tracts. The ten cycles of IBD detection were run with different thresholds for assigning IBD to the haplotypes of two individuals. The numbers varied from zero detected pairwise IBD tracts to complete IBD genomes. We empirically determined that the middle range of thresholds resulted in pairwise IBD tracts that remained stable in terms of relative number and length of detected IBD tracts between members of different pig groups. To this end, the final threshold that was used for IBD detection (5.0 −6 ) was elevated compared with that of the original paper, to allow extracting similar, but not necessarily identical, haplotypes between individuals. As the focus of this analysis was to identify regions containing haplotypes that are more similar between distantly related individuals than expected based on their inheritance, and the frequencies of similar haplotypes are leveled out, this threshold was thought to fit the data best. To estimate the frequency of shared haplotypes in different regions of the genome, the genome was divided into bins of 10,000 bp, and the number of recorded IBD tracts between the LW pigs and the two different pig groups (ASDom and EUWB) was computed per bin. As the total number of pairwise comparisons differed between the groups, these numbers were normalized, ranging from 0 (no IBD tract detected) to 1 (all individuals IBD with all individuals within the group). Relative IBD between the LW and the two competing pig groups ASDom and EUWB was then calculated by extracting per bin the normalized IBD with ASDom from the normalized IBD with EUWB. Normalized IBD for one pig group: nIBD=cIBD/tIBD (where cIBD=count of all haplotypes IBD between LW and one pig group and tIBD=total pairwise comparisons between LW and one pig group). rIBD between two pig groups: rIBD=nIBDASDom–nIBDEUWB. The distribution of rIBD for the comparison between LW-ASBr and LW-EUWB IBD haplotypes resembled and normal distribution and therefore was Z -transformed as follows: ZrIBD=(rIBD–μ)/σrIBD. Therefore, ZrIBD represents the number of s.d. that rIBD deviates from the mean rIBD. The threshold for extreme IBD with the breeds from the other continent compared with the wild boars from the same continent was set to 2 s.d. from the mean in the far right tail of the distribution. GO-enrichment analysis All annotated genes in build 10.2 (Ensembl release 67) from the S. scrofa reference genome were extracted. GO-enrichment analysis was performed for genes in the top 1.3% ( σ >2 for ZrIBD) of regions with an over-representation of ASDom haplotypes in LW pigs. The Cytoscape v.2.8.3 plugin BinGO v2.44 (ref. 44 ) was used to identify over-represented biological process-related GO terms. The human one-to-one orthologues (Ensembl db) for all pig genes were used for the analysis, as human genes are annotated more comprehensively. Significance levels were adjusted based on the Benjamini and Hochberg correction for multiple comparisons. Fst analysis To measure genetic differentiation the individuals from the Matrix were assigned to one of the following pig groups (if applicable): LW breed (LW), Asian domesticated pigs (ASDom) and European wild boar (EUWB). Pairwise Fst as described by Weir and Cockerham [20] between the LW breed and the other two groups were computed with Genepop 4.2 in bins of 10 kb over the full length of the genome [45] . Relative Fst (rFst) and Z transformation of rFst (ZrFst) were computed similarly as rIBD and ZrIBD. Correlations between ZrFst and ZrIBD values were calculated with Pearson’s product moment correlation in R. Admixture fraction To prove the existence of admixture between LW and MS in our potentially introgressed regions, but also genome-wide, we computed D -statistics [21] as implemented in qpDstats from the ADMIXTOOL software package [46] . In short, the D -statistics provide a robust test for admixture by challenging the strictly bifurcating nature of a phylogenetic tree. For a triplet of taxa P1, P2 and P3, and an outgroup O, that follows the phylogeny (((P1,P2),P3).O), one can compute the number of sites where P1 and P3 (BABA) or P2 and P3 (ABBA) share the derived state (B; assuming ancestral state, A, in the outgroup). Under a null hypothesis of no gene flow or no sub-structure (strict bifurcation), the count of ABBA and BABA should not be significantly different. Alternatively, a significant excess of either ABBA or BABA site pattern provide a conclusive proof of gene flow or sub-structure. However, as sub-structure is very unlikely to affect our analysis of domestic pigs from Asia and Europe (because of independent domestication), we can conclude that significant D implies gene flow. We computed D -statistics between LW (P1), European wild boars (P2) and Asian domestics (P3), for every possible combination of samples, using the sequence of wild boar from Sumatra as an outgroup (O). For each possible combination, we first computed a genome-wide value. Significance level was computed using a standard block jackknife, with blocks of 1 cM (assuming 1 Mb=1 cM). We also computed D -statistics in potentially admixed regions separately. Haplotype association test To examine the putative effect of the amino acid change, we used genotype data from an additional 5,143 individuals from 3 different commercial purebred lines, genotyped on the Illumina Porcine 60K iSelect Beadchip [29] for 21 markers surrounding the mutation. Line A and B are dam lines selected for reproductive traits and line C is a sire line selected for finishing traits. In all three lines, TNB was routinely recorded on sows. The EBV of the genotyped animals were obtained via routine genetic evaluation using MIXBLUP in a multitrait model [47] . The model for obtaining the EBV of TNB included fixed effects (herd-year-season, insemination number, parity, cross-fostering (Y/N), interval weaning (class)) and random effects for service sire, permanent sow and animal. Reliabilities per animal were extracted from the genetic evaluation and were based on the methodology of Tier and Meyer [48] , and animals with a reliability <0.15 were excluded from the analyses. We genotyped 64 individuals for the mutation by Sanger sequencing with the BigDye Terminator v3.1 Cycle Sequencing Kit (Applied Biosystems) on an ABI3730 sequencer. The following primers were used: AHRgene_Forward 5′-AGCAGCAGCAACAACTGTGT-3′ and AHRgene_Reverse 5′-GACACAGCTCCACCATAGCA-3′. The haplotypes, based on the 21 markers that were associated with the alleles at the site of mutation, were reconstructed. Next, all 5,143 individuals were phased with Beagle, and the G or T allele at the site of the mutation was assigned to these phased haplotypes when possible. We identified 19 unique haplotypes in the data set for which the allele at the site of mutation could be verified. The following linear model was fit to the data using R to test for a significant effect of the allele on EBV for TNB: lm(formula=EBV_TNB~LINE+Origin, weights=REL_TNB). EBV_TNB is the EBV for total number born and these values are weighted for the reliability for this trait (REL_TNB). Genetic line was included to account for differences between selection strategies between the three genetic lines A, B and C. Finally, an animal model was fit (to account for family relatedness) to the data using ASReml [49] to test for a significant effect of the allele on EBV for TNB: y = X b+ Z a+e, where b is a vector of the fixed effect for line and origin, a is the vector of the random animal genetic effect. The term e is a vector of the random residual effects assumed to be normally distributed, but weighted by the reliability of the EBV. Mutation characteristics The functional annotation of the genomic variants in the high IBD regions (σrIBD>2) was determined using Annovar [50] . The nature of the non-synonymous mutation in the gene was obtained from the webtool polyPhen 2 (ref. 51 ) by using the human orthologue AHR for the pig gene ENSSSCG00000030484 . Phylogenetics We performed our primary phylogenetic analysis using MrBayes 3.2 and our matrix of variable sites [52] . To estimate correct branch length solely from variable sites, we used the Mkv model implemented in MrBayes, which provides a likelihood framework for data sets that contains only variable characters. We recorded SNPs in four potential states (0–3). Rate of evolutions, for each SNP, were drawn from a γ -distribution. We ran two independent runs of four Marcov chain Monte Carlo (MCMC) chains with two million samples. We repeated this analysis solely based on SNPs found in the two introgressed regions on chromosome 9 and 8 separately. Extended haplotype homozygosity tests The identification of extended haplotype homozygosity was tested on 56 LW individuals that were genotyped on the Illumina Porcine 60K iSelect Beadchip [29] . First, a genome-wide scan for iHS within line was performed with the R package rehh [22] , [53] . Significance levels within line were averaged for 500 kb and correlation with the rIBD values for the same bins of 500 kb was tested with the cor.test R. Second, a reference panel of 100 individuals belonging to the Landrace, Pietrain and another LW breed was used to polarize the iHS signal in the original 56 LW individuals with the ies2rsb function in rehh [27] , [53] . To check the signal on chromosome 9, we also performed the recently developed nSL test that uses a slightly different approach to screen for extended haplotype homozygosity than the original iHS test and is robust to variation in recombination frequency [39] . The bifurcation diagram option in rehh was used to visualize the linkage disequilibrium from a focal SNP on the Beadchip that was closest to the AHR gene. Accession codes: All BAM files for the 70 re-sequenced samples have been deposited in the European Nucleotide Archive (ENA) under the accession code ERP001813 . How to cite this article: Bosse, M. et al. Genomic analysis reveals selection for Asian genes in European pigs following human-mediated introgression. Nat. Commun. 5:4392 doi: 10.1038/ncomms5392 (2014).